Increased Notch signalling inhibits anoikis and stimulates proliferation of prostate luminal epithelial cells The prostate epithelial lineage hierarchy remains inadequately defined. Recent lineage-tracing studies have implied the existence of prostate luminal epithelial progenitors with extensive regenerative capacity. However, this capacity has not been demonstrated in prostate stem cell activity assays, probably owing to the strong susceptibility of luminal progenitors to anoikis. Here we show that constitutive expression of Notch1 intracellular domain impairs secretory function of mouse prostate luminal cells, suppresses anoikis of luminal epithelial cells by augmenting NF-κB activity independent of Hes1, stimulates luminal cell proliferation by potentiating PI3K-AKT signalling, and rescues the capacities of the putative prostate luminal progenitors for unipotent differentiation in vivo and short-term self-renewal in vitro . Epithelial cell autonomous AR signalling is dispensable for the Notch-mediated effects. As Notch activity is increased in prostate cancers, and anoikis resistance is a hallmark for metastatic cancer cells, this study suggests a pro-metastatic function of Notch signalling during prostate cancer progression. Mammalian tissues consist of diverse cell types that form a defined lineage hierarchy through which tissue homeostasis is maintained and tissue repair and regeneration are executed with exquisite precision. Despite the extensive progress that has been made during the last decade, the prostate epithelial lineage hierarchy remains inadequately defined. Prostate epithelia consist of the following three types of cells: the columnar secretory luminal epithelial cells that form a continuous single layer surrounding the luminal space of prostate glands, the cuboidal basal epithelial cells that are aligned between the luminal cells and the basement membrane, and the rare neuroendocrine cells [1] . Early studies showed that prostate epithelia can regress and regenerate repeatedly in response to alternating androgen deprivation and replacement, suggesting the existence of cells that possess extensive regenerative potential [2] . Several lineage-tracing studies demonstrated that adult murine prostate basal and luminal cells are mainly self-sustained when residing in their native microenvironment under physiological conditions, suggesting the existence of stem cells or progenitors in both cell lineages [3] , [4] , [5] , [6] . The stem cell activity within the basal cell lineage has been clearly demonstrated. A fraction of human and rodent basal epithelial cells can form serially passagable, clonogenic two-dimensional (2D) holoclones or three-dimensional (3D) spheroids in vitro , implying their capacity for self-renewal [7] . In addition, when human and rodent basal prostate epithelial cells are transplanted under the renal capsules of immunodeficient mice with embryonic urogenital sinus mesenchymal (UGSM) cells, they are capable of differentiating into all three prostate epithelial lineages [8] , [9] , [10] , [11] , [12] , [13] . Finally, in several recent lineage-tracing studies, basal cells are also shown to be capable of generating luminal cells, especially in the context of prostatic inflammation [5] , [6] , [14] . In contrast, stem cells or progenitors within the luminal cell lineage remain poorly defined. Although recent lineage-tracing studies have clearly demonstrated that luminal cells residing in their native microenvironment are capable of undergoing extensive regeneration [3] , [4] , [5] , [6] , such capacity has not been recapitulated in various in vitro and in vivo assays. Unlike prostate basal cells, normal and cancerous luminal epithelial cells of both human and rodent origins rarely form colonies or spheres in 2D or 3D in vitro assays, or regenerate tissues in the prostate regeneration assay [7] , [15] . In addition, there are very few successful reports regarding the generation of immortalized normal prostate cell lines with a definitive luminal cell phenotype [16] , [17] . The failure of luminal cells to expand or regenerate in these assays was considered as a feature associated with their terminal differentiation. Nevertheless, it may also reflect their strong susceptibility to anoikis. Anoikis is apoptosis induced in cells by insufficient or inappropriate cell–matrix interactions [18] . Compared with the luminal epithelial cells, dissociated basal epithelial cells are likely more resistant to anoikis owing to several distinct intrinsic properties. First, basal cells express Bcl-2 at a higher level [19] . Second, basal cells express both adhesion-associated membrane receptors and their substrates in extracellular matrix [20] , [21] , [22] , [23] . Therefore, they are capable of establishing cell–matrix interactions cell autonomously, thereby antagonizing anoikis. Third, epithelial–mesenchymal transition has been shown to confer anoikis resistance [24] . Compared with luminal cells, basal cells display a more mesenchymal phenotype and display a gene signature that promotes epithelial–mesenchymal transition. For example, basal cells express the miR-200 family members at a lower level compared with luminal cells [25] . Finally, many growth factor receptor tyrosine kinases are preferentially expressed in basal cells versus luminal cells in normal prostate tissues [26] , [27] . Therefore, basal cells possess higher levels of steady-state activities of MAPK and AKT, which also confer anoikis resistance. The Notch signalling pathway has an important role in specifying cell fate and regulating tissue homeostasis [28] . Cross talk between Notch and nuclear factor-κB (NF-κB) has been extensively investigated, and has been shown to have important roles in tissue development and disease progression [29] . Activation of NF-κB signalling following detachment of intestinal and mammary gland epithelial cells from their native environment upregulates various anti-apoptotic pathways and has been shown to delay anoikis [23] , [30] , [31] , [32] . In this study, we show that Notch delays anoikis of prostate luminal progenitors by augmenting NF-κB activity, and rescues their capacities for short-term self-renewal and unipotent differentiation. Notch affects luminal cell growth and function in vivo Previously, we showed that an ARR2PB-Cre;ROSA(N1IC) model (hereafter referred to as PB-NICD) that expressed the Notch1 intracellular domain (NICD or N1IC) in the prostate developed prostatic intraepithelial neoplasia (PIN lesions) [33] . The prostates of PB-NICD mice were slightly heavier than those of the control ROSA(N1IC) mice (hereafter referred to as the NICD WT mice) ( Supplementary Fig. 1a,b ). PB-NICD mice developed PIN II lesions [34] with numerous micro-papillary projections containing atypical cells with hyperchromasia and a high nuclear-cytoplasmic ratio ( Fig. 1a ). There was a significant increase in epithelial proliferation as shown by Ki67 staining in Fig. 1a and Supplementary Fig.1c . Simultaneous knockout of the canonical Notch signalling transducer Rbp-J (PB-NICD-Rbp-J fl/fl triple transgenic mice) abolished the phenotypes ( Fig. 1a ), demonstrating that NICD induces luminal cell proliferation via canonical Notch signalling. Notch activation is not sufficient to transform prostate epithelial cells since PB-NICD mice did not develop adenocarcinoma even by 1.5 years of age ( Supplementary Fig. 1c ). Despite a persistently elevated proliferation index during aging, epithelial tissues that shed into the luminal space of prostate glands were frequently observed and stained positive for the cleaved Caspase 3 ( Supplementary Fig. 1c ), suggesting that Notch does not confer long-term self-renewal capacity. 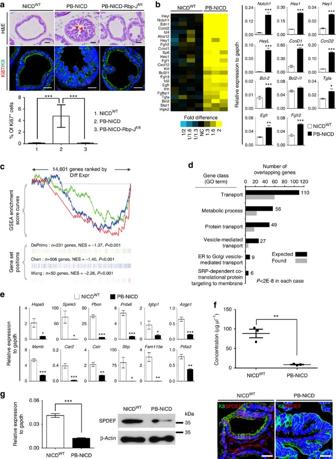Figure 1: Notch activation causes PIN lesion and impairs secretory function of prostate luminal cells. (a) H&E staining and IHC analysis of Ki67 and K8 in dorsolateral lobes of NICDWT, PB-NICD and PB-NICD-Rbp-jfl/flmouse prostates. Bar graph shows means±s.d. of percentage of Ki67+cells from 3 to 5 mice per group. Arrowheads point to micro-papillary projections. (b) Heatmap from microarray data shows upregulation of cell cycle gene ontology group in PB-NICD mouse prostates. qRT–PCR validates expression changes of representative genes in microarray analysis. (c) Gene set enrichment analysis (GSEA) shows that three independent androgen-induced gene sets are all repressed in PB-NICD mouse prostates. (d) GO analysis shows that gene ontology groups related to secretory function are downregulated in PB-NICD mouse prostates. (e) qRT–PCR validates expression changes of major secretory proteins in prostates. (f) Concentration of secretory proteins in anterior prostate lobes of 10-week-old NICDWTand PB-NICD mice. Data represent means±s.d. from three mice per group. (g) qRT–PCR, western blot and IHC analysis of SPDEF expression in NICDWTand PB-NICD mouse prostates. All qRT–PCR data represent means±s.d. from 3 to 4 mice per group. Scale bars, 25 μm. Statistical significance was calculated using thet-test (*P<0.05, **P<0.01 and ***P<0.001). Diff Expr: differential expression; ER: endoplasmic reticulum; GO: gene ontology; NES: normalized enrichment score; SRP: signal-recognition particle. Figure 1: Notch activation causes PIN lesion and impairs secretory function of prostate luminal cells. ( a ) H&E staining and IHC analysis of Ki67 and K8 in dorsolateral lobes of NICD WT , PB-NICD and PB-NICD-Rbp-j fl/fl mouse prostates. Bar graph shows means±s.d. of percentage of Ki67 + cells from 3 to 5 mice per group. Arrowheads point to micro-papillary projections. ( b ) Heatmap from microarray data shows upregulation of cell cycle gene ontology group in PB-NICD mouse prostates. qRT–PCR validates expression changes of representative genes in microarray analysis. ( c ) Gene set enrichment analysis (GSEA) shows that three independent androgen-induced gene sets are all repressed in PB-NICD mouse prostates. ( d ) GO analysis shows that gene ontology groups related to secretory function are downregulated in PB-NICD mouse prostates. ( e ) qRT–PCR validates expression changes of major secretory proteins in prostates. ( f ) Concentration of secretory proteins in anterior prostate lobes of 10-week-old NICD WT and PB-NICD mice. Data represent means±s.d. from three mice per group. ( g ) qRT–PCR, western blot and IHC analysis of SPDEF expression in NICD WT and PB-NICD mouse prostates. All qRT–PCR data represent means±s.d. from 3 to 4 mice per group. Scale bars, 25 μm. Statistical significance was calculated using the t -test (* P <0.05, ** P <0.01 and *** P <0.001). Diff Expr: differential expression; ER: endoplasmic reticulum; GO: gene ontology; NES: normalized enrichment score; SRP: signal-recognition particle. Full size image Gene expression profiling of prostate RNAs confirms that the expression of the cell cycle gene ontology group is significantly upregulated in PB-NICD prostates as compared with those of the controls, of which Notch1 and major Notch downstream targets ( Hes1, Hey1 and HeyL ), anti-apoptotic protein Bcl-2 , Cyclin D s and some growth factor receptors ( Fgfr2 and Egfr ) were verified by quantitative reverse transcription PCR (qRT–PCR; Fig. 1b ). Although the expression level of the androgen receptor (AR) was not significantly altered in PB-NICD mouse prostates ( Supplementary Fig. 1d,e ), gene set enrichment analysis revealed that the AR-induced genes from three independent data sets [35] were all significantly downregulated in PB-NICD prostates ( Fig. 1c ). This is consistent with the previous reports that Notch targets Hey1/2 and HeyL can act as AR corepressors [36] , [37] . In addition, gene ontology groups related to secretory function, such as vesicle-mediated transport, were downregulated in PB-NICD prostates ( Fig. 1d ). We confirmed by qRT–PCR that transcripts for most of the major prostate-secreted proteins [38] were drastically downregulated in PB-NICD prostates ( Fig. 1e ). In agreement with this, the concentration of secretory proteins within anterior prostate lobes of PB-NICD mice was tenfold lower than that of NICD WT mice ( Fig. 1f ). Protein secretion is an important function of terminally differentiated prostate luminal cells. Notch impairs the terminal differentiation of goblet cells in the lung and small intestine by suppressing the SAM-pointed domain-containing Ets-like factor SPDEF [39] , [40] . SPDEF was shown recently to drive mammary gland luminal cell differentiation [41] . Interestingly, SPDEF positively regulates AR transcriptional activity [42] . Figure 1g shows that Spdef was downregulated in PB-NICD mice at both the RNA and protein levels, suggesting that Notch may also impair luminal cell secretory function by negatively regulating AR activity via downregulation of SPDEF. Collectively, these studies suggest that Notch promotes proliferation of luminal epithelial cells, impairs their secretory function, but is incapable of transforming naive luminal epithelial cells. Notch promotes luminal cell survival and growth in vitro Rodent prostate epithelia are mainly composed of a single layer of cytokeratin 8 (K8)-expressing luminal cells surrounding the lumen and a discontinuous layer of cytokeratin 5 (K5)-expressing basal epithelial cells aligned between the luminal cells and the basement membrane ( Fig. 2a ). In comparison, the PIN lesions in PB-NICD mice consisted mainly of luminal cells while basal cells were significantly depleted ( Fig. 2a ). We showed previously that Notch suppressed prostate basal cell proliferation, and attributed the depletion of basal cells to the Cre activity in basal epithelial cells in the ARR2PB model [33] . 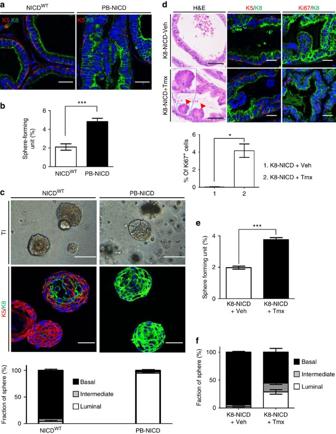Figure 2: Notch promotes formation of luminal prostate spheres. (a) IHC analysis of K5 and K8 in NICDWTand PB-NICD mouse prostates. (b) Bar graph quantifies SFUs in NICDWTand PB-NICD groups. (c) Transillumination (TI) images and IHC analysis of K5 and K8 in prostate spheres generated from NICDWTand PB-NICD mice. Bar graph quantifies types of spheres. (d) H&E staining and IHC analysis of K5, K8 and Ki67 in prostates of tamoxifen (Tmx)- and control vehicle (Veh)-treated 9-week-old K8-NICD mice. Arrowheads point to PIN I lesions. Inset shows image at higher magnification. Bar graph shows means±s.d. of percentage of Ki67+cells from three mice per group. (e,f) Bar graphs quantify SFUs and types of prostate spheres in Tmx- and Veh-treated K8-NICD groups. Data represent means±s.d. from 3 to 4 mice per group. Scale bars, 25 μm (a, fluorescent images ind); 50 μm (H&E images indand fluorescent images inc); and 100 μm (TI images inc). Statistical significance was calculated using thet-test (*P<0.05, ***P<0.001). Figure 2: Notch promotes formation of luminal prostate spheres. ( a ) IHC analysis of K5 and K8 in NICD WT and PB-NICD mouse prostates. ( b ) Bar graph quantifies SFUs in NICD WT and PB-NICD groups. ( c ) Transillumination (TI) images and IHC analysis of K5 and K8 in prostate spheres generated from NICD WT and PB-NICD mice. Bar graph quantifies types of spheres. ( d ) H&E staining and IHC analysis of K5, K8 and Ki67 in prostates of tamoxifen (Tmx)- and control vehicle (Veh)-treated 9-week-old K8-NICD mice. Arrowheads point to PIN I lesions. Inset shows image at higher magnification. Bar graph shows means±s.d. of percentage of Ki67 + cells from three mice per group. ( e , f ) Bar graphs quantify SFUs and types of prostate spheres in Tmx- and Veh-treated K8-NICD groups. Data represent means±s.d. from 3 to 4 mice per group. Scale bars, 25 μm ( a , fluorescent images in d ); 50 μm (H&E images in d and fluorescent images in c ); and 100 μm (TI images in c ). Statistical significance was calculated using the t -test (* P <0.05, *** P <0.001). Full size image When dissociated prostate epithelial cells from wild-type (WT) mice are cultured in a prostate sphere assay, only prostate basal cells are capable of forming spheroids [43] . Surprisingly, although PB-NICD mouse prostates had fewer basal cells, the sphere-forming unit (SFU) of dissociated prostate cells from PB-NICD mice was ~2.3-fold of that of NICD WT cells ( Fig. 2b ). NICD WT cells mainly generated spheres containing cells that only expressed the basal cell marker K5 (hereafter referred to as the basal prostate spheres; Fig. 2c ). A small fraction of basal spheres contained cells embedded in the centre that expressed the luminal cell marker K8, which we termed intermediate spheres. Very few spheres in the NICD WT culture were comprised solely of K8-expressing luminal cells (hereafter referred to as the luminal prostate spheres). In contrast, ~5–8% of PB-NICD spheres were basal and intermediate prostate spheres, whereas the remaining spheres were all luminal spheres ( Fig. 2c ). The luminal spheres initially appeared hollow and bright but began to fill in noticeably starting at day 4, and became morphologically similar to basal prostate spheres by the end of the assay ( Supplementary Fig. 2a ). Formation of these luminal spheres was dependent on canonical Notch signalling because prostate cells of PB-NICD-Rbp-J fl/fl triple transgenic mice did not form luminal prostate spheres ( Supplementary Fig. 2b ). Since ectopic NICD expression in basal cells does not drive their differentiation into luminal cells [33] , we reasoned that luminal prostate spheres were derived from NICD-expressing luminal cells. To directly test this hypothesis, we generated K8-CreER T2 ; ROSA(N1IC) bigenic mice (hereafter referred to as K8-NICD) with which NICD can be specifically activated in the K8-expressing luminal cells upon tamoxifen induction [44] . As shown in Fig. 2d , 3 weeks after the induction of NICD expression, K8-NICD mice developed PIN I lesions and the proliferation index of epithelial cells was markedly increased (0.03% in WT versus 4.17% in PB-NICD). We performed a prostate sphere assay using prostate cells from K8-NICD mice that have been treated with tamoxifen or vehicle control. As shown in Fig. 2e , dissociated prostate cells from tamoxifen-treated K8-NICD mice displayed a 1.9-fold increase in sphere-forming capability. The control culture contained predominantly basal prostate spheres, while both basal and luminal spheres grew out in the tamoxifen-treated K8-NICD group ( Fig. 2f ). Since tamoxifen treatment did not induce the formation of luminal spheres from NICD WT prostate cells ( Supplementary Fig. 2c ), this directly demonstrates that luminal prostate spheres are derived from NICD-expressing luminal cells. We also confirmed this conclusion using the PB-NICD model. In PB-NICD mice, prostate cells expressing NICD also express green fluorescent protein (GFP) simultaneously via an internal ribosomal entry site expressing cassette. Since Sca-1 is mainly expressed in murine prostate basal cells and stromal cells [10] , we used Sca-1 and GFP to separate luminal cells that express NICD from other cell populations ( Supplementary Fig. 2d ). Immunocytochemical analyses ( Supplementary Fig. 2e ) corroborated that expression of the basal cell markers (K5 and K14) and the luminal cell markers (K8 and AR) were enriched in Sca-1 + and Sca-1 − cells, respectively. Because stromal cells also express Sca-1, smooth muscle actin was detected in some Sca-1 + cells ( Supplementary Fig. 2h ). Individual fluorescence activated cell sorter (FACS)-isolated cell fraction was cultured in the sphere assay separately. If luminal prostate spheres are derived from Notch-expressing luminal cells, then the Sca-1 − GFP + cells should generate luminal spheres. As expected, Supplementary Fig. 2f shows that the spheres generated from the Sca-1 − cells were luminal prostate spheres, whereas Sca-1 + cells formed mostly basal prostate spheres. We also noticed the formation of luminal spheres in the Sca-1 − GFP − group, but the SFU in this population is lower compared with that of the Sca-1 − GFP + group ( Supplementary Fig. 2f ). Because the fluorescence intensity of GFP is relatively low in this mouse model, the minor sphere-forming activity from the Sca-1 − GFP − group may be attributed by the contaminated Sca-1 − GFP + cells during cell sorting. These results further corroborate that luminal prostate spheres were generated by NICD-expressing luminal cells. Interestingly, only 4.5% NICD-expressing luminal cells can survive and proliferate in vitro in response to Notch ( Supplementary Fig. 2g ). Similar observation was made when Lin − Sca-1 − CD49f low luminal cells were used in the prostate sphere assay ( Supplementary Fig. 2i ). These sphere-forming luminal cells may be functionally distinct from the Notch-expressing luminal cells that did not form spheres and may represent the putative prostate luminal progenitors. Notch rescues prostate luminal progenitor activity Previous studies showed that FACS-isolated luminal cells from intact mice were incapable of regenerating prostate tissues in a transplantation-based prostate regeneration assay [8] , [9] . Since Notch promotes survival and proliferation of luminal cells in the prostate sphere assay, we hypothesized that increased Notch activity might promote the in vivo survival of dissociated prostate luminal progenitors and rescue their regenerative capability in the prostate regeneration assay. Sca-1 + (basal and stromal cells) and Sca-1 − (luminal cells) cells were FACS isolated from WT and PB-NICD mice. CD49f was not used during the sorting since Sca-1 is sufficient to separate luminal cells. Immunocytochemical analysis of specific lineage markers confirmed the identities of the FACS-sorted cells ( Supplementary Fig. 2e ). Each cell fraction was mixed with urogenital sinus mesenchyme cells separately and incubated subcutaneously in immunodeficient male mice to allow regeneration. As shown in Fig. 3a , NICD WT Sca-1 + cells generated the typical prostatic glandular structures comprising K5 + P63 + basal cells and K8 + AR + luminal cells [10] . PB-NICD Sca-1 + cells generated similar structures but the gland-forming unit was lower than that of NICD WT cells (0.03% in WT group versus 0.015% in PB-NICD group), consistent with our previous study showing that Notch activity suppresses basal stem cell activity [33] . In addition, glands generated in the PB-NICD group often contained less eosinophilic secretions in luminal spaces ( Fig. 3a ), suggesting potential defects in secretory function of luminal epithelial cells. As expected, NICD WT Sca-1 − luminal cells failed to regenerate discernible glandular structures ( Fig. 3b ). In contrast, Sca-1 − luminal cells from PB-NICD mice regenerated tissues containing small glandular structures made solely of K8 + luminal cells that expressed AR ( Fig. 3b ). Many glands contained multiple layers of cells resembling the histopathology observed in the PB-NICD model. The average luminal gland-forming unit was ~0.3%. It should be noted that the estimated glandular-forming units represent the minimal values because we enumerated the numbers of the glandular structures from tissue sections that contained tissue specimens with the largest diameter instead of reconstructed 3D images. These results show that NICD can promote the in vivo survival and proliferation of a small fraction of prostate luminal cells in the regeneration assay. This is consistent with the fact that only a small fraction of NICD-expressing luminal cells can survive and proliferate in vitro in the sphere assay, and further implies a primitive lineage hierarchical status of these cells within the luminal cell lineage. 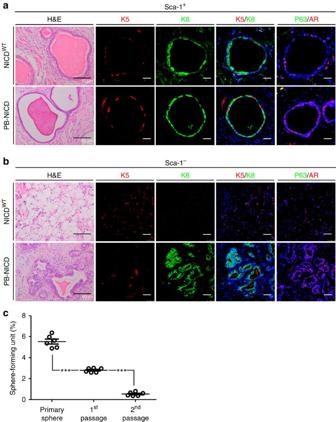Figure 3: Notch rescues the capacities of dissociated luminal progenitors for unipotent differentiation and short-term self-renewal. (a,b) H&E staining and IHC analysis of K5, K8, AR and P63 in tissues regenerated from Sca-1+and Sca-1−cells of NICDWTand PB-NICD mice. (c) Sphere-forming activity of serially passaged luminal sphere cultures. Scale bars, 25 μm (fluorescent images ina); 50 μm (fluorescent images inb); and 100 μm (H&E images ina,b).Data represent means±s.d. from three independent experiments. Statistical significance was calculated using thet-test (***P<0.001). Figure 3: Notch rescues the capacities of dissociated luminal progenitors for unipotent differentiation and short-term self-renewal. ( a , b ) H&E staining and IHC analysis of K5, K8, AR and P63 in tissues regenerated from Sca-1 + and Sca-1 − cells of NICD WT and PB-NICD mice. ( c ) Sphere-forming activity of serially passaged luminal sphere cultures. Scale bars, 25 μm (fluorescent images in a ); 50 μm (fluorescent images in b ); and 100 μm (H&E images in a , b ).Data represent means±s.d. from three independent experiments. Statistical significance was calculated using the t -test (*** P <0.001). Full size image To determine whether NICD-expressing luminal sphere-forming cells possess self-renewal capacity, we examined whether luminal prostate spheres can be serially passaged. Prostate spheres were enzymatically dissociated into single cells and replated to form secondary and tertiary spheres. As shown in Fig. 3c , primary luminal spheres can be passaged twice but the SFU decreased markedly. This result suggests that luminal sphere-forming cells only possess limited self-renewal capacity. β-Catenin is not required for luminal sphere formation Basal prostate sphere cells possess long-term self-renewal capability in vitro [43] . To gain insights into how and why NICD-expressing prostate luminal cells can survive and proliferate in vitro only for short term, we compared protein expression profiles of the luminal and the basal prostate spheres using a reverse-phase protein array (RPPA) containing 170 different antibodies. The RPPA analysis shows that luminal prostate sphere cells expressed higher levels of several signalling components of the Wnt pathway including β-catenin, among which we confirmed by Western blot the expression of β-catenin ( Supplementary Fig. 3a,b ). We generated PB-Cre;Catnb lox(ex3) bigenic mice that express a stabilized β-catenin specifically in the prostate epithelia [45] . Dissociated prostate cells from PB-Cre; Catnb lox(ex3) mice did not form luminal prostate spheres in vitro ( Supplementary Fig. 3c,d ), suggesting that expression of β-catenin in prostate luminal cells is not sufficient to promote their in vitro survival. In addition, C57Bl/6 mouse prostate luminal cells infected with the lentivirus expressing a high level of constitutively active β-catenin driven by the human ubiquitin promoter also failed to form luminal spheres in vitro ( Supplementary Fig. 3e,f ). This excludes the possibility that the failure of PB-Cre; Catnb lox(ex3) cells to generate luminal prostate spheres is due to insufficient expression of stabilized β-catenin driven by the endogenous promoter. To determine whether β-catenin is essential for luminal sphere formation, we expressed a dominant-negative β-catenin (dN-βCatenin) [46] in the luminal prostate epithelial cells of PB-NICD mice. Expression of dN-βCatenin suppressed the Wnt target c-Myc ( Supplementary Fig. 3g ), but did not inhibit sphere formation or reduce sphere size ( Supplementary Fig. 3h–j ). Collectively, these results show that the transcriptional activity of β-Catenin is neither sufficient nor essential for the survival and proliferation of luminal sphere cells. PI3K-AKT is necessary for luminal sphere cell proliferation The RPPA assay also revealed that NICD WT basal prostate sphere cells possess a higher level of mammalian target of rapamycin (mTOR) activity, although PB-NICD luminal sphere cells expressed a relatively higher level of pAKT probably due to Notch-mediated transcriptional repression of Pten [47] ( Fig. 4a ). This is probably because basal cells express various growth factor receptor kinases hence may have more signal entry and feedback inputs [26] , [27] . Western blot analysis confirmed the differential expression levels of several major signalling components ( Fig. 4b ). This difference in mTOR activity may partially explain why basal prostate sphere cells can proliferate extensively in vitro . 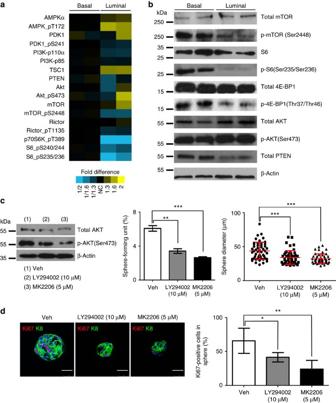Figure 4: PI3K-AKT signalling is necessary for proliferation of luminal prostate sphere cells. (a) Heatmap from RPPA analysis shows that basal sphere cells possess higher mTOR activity. (b) Western blot validates expression of several major PI3K-AKT-mTOR signalling components in basal and luminal prostate spheres. Individual lanes represent independent samples. (c) Western blot shows that LY294002 and MK2206 suppress AKT activity. Bar and dot graphs quantify sphere-forming activity and prostate sphere size from three independent experiments. (d) IHC analysis of Ki67 and K8 in luminal prostate spheres treated with vehicle (Veh), LY294002 and MK2206. Bar graph shows quantification. Data represent means±s.d. from three independent experiments. Scale bars, 25 μm. Statistical significance was calculated using thet-test (*P<0.05, **P<0.01 and ***P<0.001). PTEN: phosphatase and tensin homolog. Figure 4: PI3K-AKT signalling is necessary for proliferation of luminal prostate sphere cells. ( a ) Heatmap from RPPA analysis shows that basal sphere cells possess higher mTOR activity. ( b ) Western blot validates expression of several major PI3K-AKT-mTOR signalling components in basal and luminal prostate spheres. Individual lanes represent independent samples. ( c ) Western blot shows that LY294002 and MK2206 suppress AKT activity. Bar and dot graphs quantify sphere-forming activity and prostate sphere size from three independent experiments. ( d ) IHC analysis of Ki67 and K8 in luminal prostate spheres treated with vehicle (Veh), LY294002 and MK2206. Bar graph shows quantification. Data represent means±s.d. from three independent experiments. Scale bars, 25 μm. Statistical significance was calculated using the t -test (* P <0.05, ** P <0.01 and *** P <0.001). PTEN: phosphatase and tensin homolog. Full size image We reasoned that PB-NICD luminal sphere cells are capable of proliferating in vitro partly because they possess a higher PI3K-AKT activity than NICD WT luminal cells. This hypothesis is supported by the fact that the gene signature upregulated by AKT [48] was enriched in prostate tissues of PB-NICD mice compared with WT mice (57 shared genes, one-sided Fisher’s exact test, P =3.7e−10; Supplementary Fig. 4 ). Consistently, treating PB-NICD prostate sphere culture with the PI3K inhibitor LY294002 efficiently reduced AKT phosphorylation, suppressed luminal prostate sphere-forming activity by 45% and reduced sphere diameter by 33% ( Fig. 4c ). Loss of function of Pten is not sufficient to confer anoikis resistance on luminal cells, because Pten-null prostate luminal cells are incapable of forming luminal prostate spheres in vitro [49] . Therefore, LY294002 treatment may not directly impinge on the survival of prostate sphere-forming cells, but attenuates the sphere-forming activity by suppressing cell proliferation. Ki67 staining confirmed that LY294002 attenuated proliferation of luminal prostate sphere cells ( Fig. 4d ). Similarly, the AKT inhibitor MK2206 reduced AKT activity, suppressed luminal prostate sphere-forming activity by 57% and reduced sphere diameter by 37%, and inhibited cell proliferation as measured by Ki67 staining ( Fig. 4c,d ). These results show that the PI3K-AKT signalling is necessary for the in vitro proliferation of luminal prostate sphere cells. Notch mediates anti-apoptotic signalling via NF-κB The RPPA assay also revealed that luminal sphere cells expressed phosphor-Ser 536 P65 at a higher level ( Fig. 5a ). In addition, the expression levels of both pro-apoptotic and anti-apoptotic proteins were higher in the luminal sphere cells, suggesting an intense balance between the survival and apoptosis signals. Western blot analysis confirmed that luminal prostate sphere cells expressed higher levels of phosphorylated P65 as well as several direct NF-κB target genes such as Bcl-2, Bcl-xL and cIAP1 ( Fig. 5b ). The transcriptional activity of phosphorylated P65 can be affected by both nuclear localization and DNA binding. To determine definitively whether NICD-expressing luminal prostate sphere cells possess a high level of NF-κB activity, we bred PB-NICD mice with an NF-κB-dependent in vivo luciferase reporter strain from Taconic (NF-κB-RE-Luc). 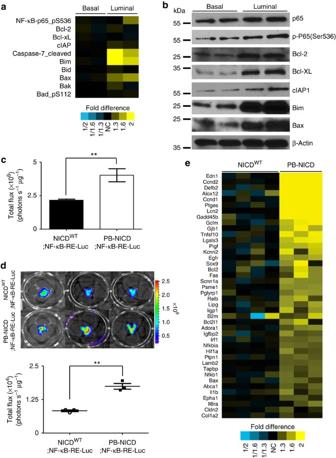Figure 5: Notch augments NF-kB activity in prostate luminal cells. (a) Heatmap from RPPA analysis shows that luminal sphere cells express higher levels of phosphorylated P65 and proteins regulating apoptosis. (b) Western blot validates expression of representative proteins in RPPA assay. Individual lanes represent independent samples. (c) Bioluminescence assay of NF-κB activity in basal spheres generated from NICDWTmice and luminal spheres from PB-NICD mice. Bar graph shows means±s.d. from three independent experiments. (d) Bioluminescence assay of NF-κB activity in 10-week-old NICDWT; NF-κB-RE-Luc and PB-NICD;NF-κB-RE-Luc mice. Dot graph shows means±s.d. from three pairs of mice. (e) Heatmap from microarray data shows upregulation of representative NF-κB target genes in PB-NICD mouse prostates. Statistical significance was calculated using thet-test (**P<0.01). Figure 5c showed that the bioluminescence signal of prostate sphere cells (95% of which were luminal spheres) derived from PB-NICD;NF-κB-RE-Luc mice was 1.9-fold higher than that of the basal spheres derived from age-matched control NICD WT ;NF-κB-RE-Luc mice. Since NICD expression in basal spheres did not affect NF-κB activity ( Supplementary Fig. 5 ), these results demonstrate that luminal sphere cells possess a higher NF-κB activity than basal sphere cells. The increased NF-κB activity in luminal cells is induced by NICD because the bioluminescence signal in the prostates of PB-NICD;NF-κB-RE-Luc mice is 2.1-fold that of the prostates in control NICD WT ;NF-κB-RE-Luc mice ( Fig. 5d ). Finally, many known NF-κB-regulated genes ( http://www.nf-kb.org ) were enriched in the genes upregulated in the PB-NICD group as compared with the control (26 shared genes, one-sided Fisher’s exact test, P =1.00e−6). Figure 5e shows some representative NF-κB target genes that were upregulated in the PB-NICD group. Of note, both NF-κb1 and Relb were upregulated. This further corroborates that Notch promotes NF-κB activity in prostate luminal cells. Figure 5: Notch augments NF-kB activity in prostate luminal cells. ( a ) Heatmap from RPPA analysis shows that luminal sphere cells express higher levels of phosphorylated P65 and proteins regulating apoptosis. ( b ) Western blot validates expression of representative proteins in RPPA assay. Individual lanes represent independent samples. ( c ) Bioluminescence assay of NF-κB activity in basal spheres generated from NICD WT mice and luminal spheres from PB-NICD mice. Bar graph shows means±s.d. from three independent experiments. ( d ) Bioluminescence assay of NF-κB activity in 10-week-old NICD WT ; NF-κB-RE-Luc and PB-NICD;NF-κB-RE-Luc mice. Dot graph shows means±s.d. from three pairs of mice. ( e ) Heatmap from microarray data shows upregulation of representative NF-κB target genes in PB-NICD mouse prostates. Statistical significance was calculated using the t -test (** P <0.01). Full size image NF-κB signalling is essential for the in vitro survival of luminal prostate sphere-forming cells because the NF-κB inhibitor BAY-11-7085 suppressed P65 phosphorylation and luminal sphere-forming activity in a dosage-dependent manner ( Fig. 6a ). WT basal prostate sphere cells also succumbed to NF-κB inhibition ( Supplementary Fig. 6a ). In addition, ectopic expression of a degradation-resistant super IκBα in PB-NICD luminal cells suppressed their sphere-forming activity markedly ( Fig. 6b ), corroborating that NF-κB is essential for the survival of luminal prostate sphere-forming cells in vitro . 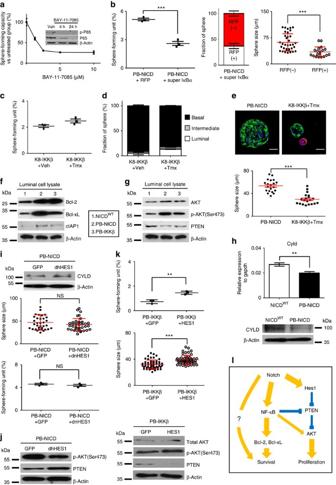Figure 6: Notch delays anoikis and promotes proliferation by augmenting NF-κB activity. (a) Inhibition of luminal prostate sphere formation by BAY-11-7085. Inset image: western blot analysis of pho-P65. (b) Super IκBα suppresses luminal sphere formation. Data represent means±s.d. from three independent experiments. (c,d) Quantitation of SFUs (c) and prostate sphere types (d) from prostate cells of K8-IKKβ mice treated with tamoxifen (Tmx) and vehicle (Veh). Data represent means±s.d. from three independent experiments. (e) Comparison of sizes of PB-NICD and K8-IKKβ luminal prostate spheres. Dot graph shows means±s.d. from one of the two independent experiments. Scale bars, 25 μm. (f) Western blot of expression of Bcl-2, Bcl-xL and cIAP1 in FACS-sorted prostate luminal cells from WT, PB-NICD and PB-IKKβ mice. (g) Western blot of Pten expression and AKT activity in FACS-sorted prostate luminal cells from WT, PB-IKKβ and PB-NICD mice. (h) qRT–PCR and Western blot of cylindromatosis (Cyld) expression in NICDWTand PB-NICD mouse prostates. qRT–PCR data represent means±s.d. from three independent experiments. (i) Expression of dominant-negative Hes1 (dN-Hes1) in PB-NICD cells upregulates Cyld expression but does not significantly affect luminal sphere formation and size. Dot graphs show data representing means±s.d. from three independent experiments. (j) Western blot analysis of Pten expression and AKT activity in luminal spheres derived from PB-NICD cells infected by GFP and dN-Hes1 lentivirus. (k) Ectopic expression of Hes1 in FACS-sorted PB-IKKβ prostate luminal cells enhances AKT activity and increases luminal SFU and sphere size. Dot graphs show data representing means±s.d. from three independent experiments. (l) Schematic illustration of molecular mechanism through which Notch and NF-κB promote formation of luminal spheres. Boldness of arrow line reflects signalling contribution. Statistical significance was calculated using thet-test (**P<0.01, ***P<0.001). NS, not significant. PTEN: phosphatase and tensin homolog; RFP: red fluorescence protein. Figure 6: Notch delays anoikis and promotes proliferation by augmenting NF-κB activity. ( a ) Inhibition of luminal prostate sphere formation by BAY-11-7085. Inset image: western blot analysis of pho-P65. ( b ) Super IκBα suppresses luminal sphere formation. Data represent means±s.d. from three independent experiments. ( c , d ) Quantitation of SFUs ( c ) and prostate sphere types ( d ) from prostate cells of K8-IKKβ mice treated with tamoxifen (Tmx) and vehicle (Veh). Data represent means±s.d. from three independent experiments. ( e ) Comparison of sizes of PB-NICD and K8-IKKβ luminal prostate spheres. Dot graph shows means±s.d. from one of the two independent experiments. Scale bars, 25 μm. ( f ) Western blot of expression of Bcl-2, Bcl-xL and cIAP1 in FACS-sorted prostate luminal cells from WT, PB-NICD and PB-IKKβ mice. ( g ) Western blot of Pten expression and AKT activity in FACS-sorted prostate luminal cells from WT, PB-IKKβ and PB-NICD mice. ( h ) qRT–PCR and Western blot of cylindromatosis (Cyld) expression in NICD WT and PB-NICD mouse prostates. qRT–PCR data represent means±s.d. from three independent experiments. ( i ) Expression of dominant-negative Hes1 (dN-Hes1) in PB-NICD cells upregulates Cyld expression but does not significantly affect luminal sphere formation and size. Dot graphs show data representing means±s.d. from three independent experiments. ( j ) Western blot analysis of Pten expression and AKT activity in luminal spheres derived from PB-NICD cells infected by GFP and dN-Hes1 lentivirus. ( k ) Ectopic expression of Hes1 in FACS-sorted PB-IKKβ prostate luminal cells enhances AKT activity and increases luminal SFU and sphere size. Dot graphs show data representing means±s.d. from three independent experiments. ( l ) Schematic illustration of molecular mechanism through which Notch and NF-κB promote formation of luminal spheres. Boldness of arrow line reflects signalling contribution. Statistical significance was calculated using the t -test (** P <0.01, *** P <0.001). NS, not significant. PTEN: phosphatase and tensin homolog; RFP: red fluorescence protein. Full size image To investigate whether enhanced NF-κB signalling is sufficient to promote in vitro survival and proliferation of prostate luminal cells, we took advantage of a K8-CreER T2 ;Rosa26-LSL-IKKβ Ca bigenic model (hereafter referred to as K8-IKKβ). Upon tamoxifen treatment, the constitutively activated IKKβ was specifically expressed in the K8-expressing prostate luminal cells. As shown in Figure 6c , IKKβ activation did not substantially increase sphere-forming activity, but did promote the formation of luminal sphere cells (5.3 versus 13.1%) ( Fig. 6d ). Of note, the size of the K8-IKKβ luminal spheres was smaller than that of the PB-NICD luminal spheres ( Fig. 6e ). Similar observations were made when the ARR2PB-Cre; Rosa26-LSL-IKKβ Ca bigenic mice were examined ( Supplementary Fig. 6b,c ). No obvious phenotype was observed in PB-IKKβ and K8-IKKβ mice, consistent with a previous study showing that IKKβ alone is insufficient for transformation [50] . Collectively, these results demonstrate that increased NF-κB activity in prostate luminal cells is sufficient to delay anoikis of luminal sphere-forming cells. However, NF-κB is less potent than Notch, suggesting that Notch signalling mediates additional NF-κB-independent signalling to antagonize anoikis and promote proliferation of luminal sphere-forming cells. NF-κB promotes the in vitro survival of luminal cells by upregulating anti-apoptotic proteins. The expression levels of the NF-κB target genes Bcl-2, Bcl-xL and cIAP1 in prostate lysates were all upregulated in the FACS-sorted luminal cells from the PB-IKKβ and PB-NICD models as compared with WT mice ( Fig. 6f ). NF-κB has also been shown to suppress Pten expression [51] and increase AKT expression or activity [52] . However, downregulation of Pten and increased AKT activity in PB-IKKβ mice compared with WT mice was not as significant as that seen in PB-NICD mice ( Fig. 6g ). This may partly explain why the size of luminal prostate spheres in PB-IKKβ group was smaller than that of the PB-NICD group. Notch is capable of enhancing NF-κB activity by a Hes1-dependent mechanism (Hes1-mediated suppression of Cyld , a deubiquitinase that negatively regulates the IKK complex) [53] and Hes1-independent mechanisms (NICD-induced expression of NF-κB, NICD-enhanced IKKα activity, or NICD-mediated NF-κB nuclear retention) [54] , [55] , [56] . Cyld was indeed downregulated at both the RNA and protein levels in prostate tissues of PB-NICD mice ( Fig. 6h ). While ectopic expression of a dN-Hes1 upregulated Cyld expression, luminal sphere-forming activity was not affected ( Fig. 6i ), suggesting that Hes1-mediated Cyld suppression does not play a role in NF-κB-mediated survival of luminal prostate sphere-forming cells. The size of luminal spheres was slightly reduced though the change did not reach statistical significance ( P =0.06; Fig. 6i ), which implies that Hes1 may regulate the proliferation of luminal sphere cells. This implication is supported by the observation that ectopic expression of dN-Hes1 slightly increased Pten expression and reduced AKT activity in PB-NICD luminal sphere cells ( Fig. 6j ). In addition, ectopic expression of Hes1 increases the SFU of FACS-sorted luminal cells of PB-IKKβ mice as well as the size of the generated luminal prostate spheres ( Fig. 6k ). The increased sphere size indicates that Hes1-mediated signalling cooperates with NF-κB to promote proliferation, as corroborated by increased AKT activity ( Fig. 6k ). On the other hand, we believe that increased SFU is not a direct effect of Hes1 on the survival of luminal sphere-forming cells since ectopic Hes1 expression in WT prostate luminal cells was not sufficient to induce the formation of luminal prostate spheres in vitro ( Supplementary Fig. 6d,e ). Instead, the increased SFU reflects enhanced proliferation of some PB-IKKβ luminal progenitors that are otherwise incapable of doing so in the absence of Hes1-mediated growth signalling. Collectively, as schematically illustrated in Fig. 6l , our study demonstrates that Notch confers anoikis resistance to luminal prostate sphere-forming cells through Hes1-independent NF-κB activation and probably also through some other unidentified signalling, while optimal proliferation of luminal sphere cells relies on an elevated activity of AKT regulated by both NF-κB and Hes1. Epithelial AR is dispensable for luminal sphere formation Luminal sphere-forming cells propagate in vitro without testosterone, and their proliferation is not affected by addition of di-hydro-testosterone ( Supplementary Fig. 7 ). It was difficult to conclude via immunohistochemistry (IHC) analysis whether these cells completely lacked expression of the AR and its ligand-independent truncated isoforms or expressed them at very low levels. To determine definitively whether AR is essential for the survival and proliferation of luminal sphere-forming cells, we eliminated epithelial AR in the PB-NICD model by generating ARR2PB-Cre;ROSA(N1IC);AR fl/Y triple transgenic mice (PB-NICD-AR KO ). The prostates of PB-NICD-AR KO mice were half the weight of PB-NICD prostates, but haematoxylin and eosin (H&E) staining showed that both models developed PIN lesions with similar dynamics ( Fig. 7a,b ). AR was efficiently knocked out in the majority of prostate epithelial cells ( Fig. 7c ). The epithelial cells in the PIN lesions of the two models proliferated at a similar rate, but the apoptosis index in the PB-NICD-AR KO group was 3.1-fold higher ( Fig. 7d,e ). These results indicate that AR is not essential for the NICD-mediated mitogenic signalling, but positively regulates the survival of luminal epithelial cells. Dissociated prostate cells from PB-NICD-AR KO and PB-NICD mice were cultured in the sphere assay. 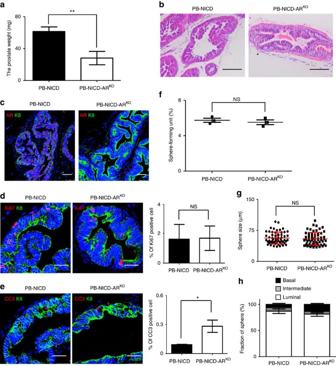Figure 7: Epithelial AR is dispensable for NICD-induced survival and proliferation of luminal sphere-forming cells. (a) Bar graph quantifies weight of 9-week-old PB-NICD and PB-NICD-ARKOmouse prostates. Data represent means±s.d. from four pairs of mice. (b) H&E staining of 9-week-old PB-NICD and PB-NICD-ARKOmouse prostates. (c) IHC analysis of AR in PB-NICD and PB-NICD-ARKOmouse prostates. (d,e) IHC analyses of Ki67 and cleaved caspase 3 in PB-NICD and PB-NICD-ARKOmouse prostates. Bar graphs show means±s.d. from three mice per group. (f–h) Bar and dot graphs quantify SFUs, sphere size and types in PB-NICD and PB-NICD-ARKOgroups. Scale bars, 100 μm (a); 50 μm (c); and 25 μm (d,e). Dot and bar graphs show data representing means±s.d. from three independent experiments. Statistical significance was calculated using thet-test (*P<0.05, **P<0.01). NS, not significant. Figure 7f–h showed that sphere-forming units, sphere size and the percentage of luminal spheres were all similar between the cultures of the two groups, demonstrating that epithelial AR signalling is dispensable for the in vitro survival and proliferation of luminal sphere-forming cells. Figure 7: Epithelial AR is dispensable for NICD-induced survival and proliferation of luminal sphere-forming cells. ( a ) Bar graph quantifies weight of 9-week-old PB-NICD and PB-NICD-AR KO mouse prostates. Data represent means±s.d. from four pairs of mice. ( b ) H&E staining of 9-week-old PB-NICD and PB-NICD-AR KO mouse prostates. ( c ) IHC analysis of AR in PB-NICD and PB-NICD-AR KO mouse prostates. ( d , e ) IHC analyses of Ki67 and cleaved caspase 3 in PB-NICD and PB-NICD-AR KO mouse prostates. Bar graphs show means±s.d. from three mice per group. ( f – h ) Bar and dot graphs quantify SFUs, sphere size and types in PB-NICD and PB-NICD-AR KO groups. Scale bars, 100 μm ( a ); 50 μm ( c ); and 25 μm ( d , e ). Dot and bar graphs show data representing means±s.d. from three independent experiments. Statistical significance was calculated using the t -test (* P <0.05, ** P <0.01). NS, not significant. Full size image Previous studies have suggested that Notch signalling may have an important role in prostate cancer progression. Notch activity has been shown to be increased in prostate cancer especially in advanced metastatic disease, although some cellular biological studies suggested otherwise [57] . More interestingly, Notch activity is higher in metastatic prostate tumour specimens than in primary tumour specimens [58] , [59] . Notch activity is enriched in the putative prostate cancer stem cells [60] and docetaxol-resistant prostate tumour cells [61] . Our study in mouse models showed that increased Notch activity drives luminal epithelial proliferation and causes the formation of PIN lesions. More importantly, NICD confers anoikis resistance to dissociated luminal cells. Anoikis resistance is a hallmark for metastatic cancer cells. Therefore, our study supports a potential role of Notch in prostate cancer metastasis. In addition, we showed that Notch confers anoikis resistance to the putative luminal progenitor cells through activation of NF-κB signalling, which is also consistent with a previous study showing that prostate tumour-initiating stem-like cells exhibited increased NF-κB signalling [62] . Several lines of evidence support the existence of a hierarchy within the luminal cell lineage. First, luminal cells are phenotypically heterogeneous. For example, they express varying levels of important transcription factors such as NKX3.1 (ref. 63 ). Second, luminal cells behave differentially in response to androgen deprivation. Although the majority of luminal cells succumb to androgen deprivation, some luminal cells can survive. Third, only some luminal epithelial cells possess the capacity to retain a bromodeoxyuridine label [64] . Finally, recent in vivo lineage-tracing studies have demonstrated the capability of the luminal lineage to self-sustain [3] , [4] , [5] , [6] . However, phenotypic and molecular features of these cells remain largely unknown. This is mainly due to a lack of in vitro or in vivo experimental systems through which the progenitor activity can be assayed quantitatively. We showed that only a consistently small fraction of NICD-expressing luminal epithelial cells are capable of forming luminal spheres in vitro and generate glandular structures in vivo . These observations suggest that these cells possess the capacities for short-term self-renewal and unipotent differentiation, and imply that they are intrinsically distinct from those that are incapable of forming spheres or glands. Ectopic Notch activity promotes survival signalling partly by augmenting NF-κB, hence enabling their short-term in vitro propagation. We reason that these NICD-expressing luminal sphere-forming cells may represent the putative luminal progenitors or transit-amplifying/intermediate cells [65] , which probably constitute at least 4.5% of luminal cells based on our study. It is likely that the sphere-forming cells in vitro are the same cells that regenerate luminal glandular structures in vivo , which should be able to be directly interrogated once these cells are phenotypically characterized. A more compelling and direct approach to characterize prostate luminal progenitors would be to physically isolate these cells, and show that they possess progenitor activity in the presence of anti-anoikis signalling. As an attempt of this approach, we have prepared dissociated WT prostate luminal cells and infected them with lentivirus-expressing NICD. However, they failed to generate luminal prostate spheres efficiently. This observation implies that anoikis is initiated immediately after cell dissociation. Therefore, the anti-anoikis and pro-proliferative signalling may have to be present before cell dissociation in order for these cells to survive and expand in vitro . Transgenic mouse models that harbour CreER transgene driven by specific promoters in conjunction with the ROSA-LSL-NICD model may be used in the future to further determine the phenotypic identity of prostate luminal progenitors. It should be noted that our observation that Notch signalling confers anoikis resistance to some luminal epithelial cells does not imply that Notch signalling is essential for the maintenance of the luminal progenitors in vivo . Nor does it imply that luminal prostate epithelial cells possessing active Notch signalling in WT mice are the luminal progenitors. An interesting feature of luminal sphere cells is that they do not express AR or express AR at a very low level. In addition, AR is not essential for the survival and proliferation of luminal sphere-forming cells. These features resemble those of the putative prostate cancer stem cells that do not express AR or PSA [62] , [66] , [67] , [68] . These similarities imply that these luminal progenitors may serve as one of the origins for prostate cancer stem cells. Therefore, future phenotypic and molecular characterization of these cells will also provide novel insights into the properties and identities of prostate cancer stem cells. Mice All animals used in this study received humane care in compliance with the regulations relating to animals and experiments involving animals and adheres to principles stated in the Guide for the Care and Use of Laboratory Animals, NIH Publication, 1996 edn, and the protocol was approved by the Institutional Animal Care Committee of Baylor College of Medicine. The C57BL/6 and NOD/SCID mice were purchased from Charles River (Wilmington, MA). The Gt(ROSA)26Sor tm1(Notch1)Dam/J (ICNf/f) , and B6(Cg)- Gt(ROSA)26Sor tm4(Ikbkb)Rsky /J mice were purchased from the Jackson Laboratory (Bar Harbor, ME). The NF-kB-RE-Luc mice were purchased from Taconic (Hudson, NY). The ARR2PB-Cre transgenic mice were from Dr Fen Wang at the Institute of Bioscience and Technology, Texas A&M Health Science Center. The K8-CreER T2 mice were generated by our laboratory [44] . The RBP-J f/f mice were obtained from Dr Tasuku Honjo at Kyoto University. The AR f/Y mice were generated by Drs Guido Verhoeven and Karel De Gendt, and were internally transferred from the laboratory of Dr Alexander Agoulnik at Baylor College of Medicine [69] . The Catnb lox(ex3) mice were internally transferred from the laboratory of Dr David Spencer at Baylor College of Medicine. Mice were genotyped by PCR using mouse genomic DNA from tail biopsy specimens. The sequences of genotyping primers and the expected band sizes for PCR are listed in Supplementary Table 1 . PCR products were separated electophoretically on 1% agarose gels and visualized via ethidium bromide under UV light. Tamoxifen treatment Tamoxifen (Sigma-Aldrich, St Louis, MO) was dissolved into corn oil and was administrated intraperitoneally into experimental mice at the age of 8 weeks (2–5 mg per 40 g per day for 4 consecutive days). Lentivirus generation and infection cDNA encoding Hes1 and dN-Hes1 were purchased from Addgene (cat. nos. 17624 and 24982; Cambridge, MA). cDNAs encoding constitutively activated β-Catenin and dN-βCatenin [46] were obtained from Drs Roger Lo and Pierre McCrea, respectively. These cDNAs were PCR amplified, verified by sequencing and cloned into the FU-CGW or FU-CRW lentiviral vectors [70] using the Eco RI or Xba I sites. Dissociated prostate cells were infected by lentivirus at 1,500 g for 90 min at 25 °C (ref. 70 ). Prostate sphere and prostate regeneration assays Prostate tissues were digested in Dulbecco's modified eagle medium (DMEM)/F12/collagenase/hyaluronidase/FBS (StemCell Technologies, Vancouver, Canada) for 3 h at 37 °C, followed by an additional digestion in 0.25% Trypsin-EDTA (Invitrogen, Carlsbad, CA) on ice for 1 h. Subsequently, digested cells were suspended in Dispase (Invitrogen; 5 mg/ml) and DNase I (Roche Applied Science, Indianapolis, IN; 1 mg ml −1 ), and pipetted vigorously to dissociate cell clumps. Dissociated cells were then passed through 70 μm cell strainers (BD Biosciences, San Jose, CA) to get single cells. Prostate sphere assays and prostate regeneration assays were performed using cells from 7–12-week-old male experimental mice [10] , [43] . In the prostate sphere assay, 1–2 × 10 4 dissociated prostate cells were cultured in 1:1 Matrigel/PrEGM (Matrigel (BD Biosciences, San Jose, CA)/PrEGM (Lonza, Walkersville, MD)). Prostate spheres were defined as spheroids with a diameter >25 μm after a 6-day culture. In the prostate regeneration assay, 1 × 10 4 to 1 × 10 5 dissociated cells or FACS-sorted cells were mixed with 1 × 10 5 mouse urogenital sinus mesenchyme cells and resuspended in transplantation solution (PrEGM media (Lonza):Matrigel (BD Biosciences, San Jose, CA), 1:1 (v/v)). Cell mixtures were injected subcutaneously into 10-week-old male NOD/SCID mice and incubated for 8 weeks. To semi-quantitate the number of glandular structures generated in the prostate regeneration assay, we enumerated the numbers of the glandular structures from tissue sections that contained tissue specimens with the largest diameter. Since we were not able to reconstruct the regenerated tissue in three dimensions, the estimated glandular-forming units should represent the minimal values. Collection of prostatic secretions Dissected anterior prostate lobes were cut into halves using syringe needles and prostate secretions were squeezed out by centrifugation at 6,000 g for 1 min. Protein concentrations were determined by a Bradford Assay kit (Bio-Rad, Hercules, CA). Pharmacological manipulation of signalling pathways LY294002, MK2206 and BAY-11-7085 were purchased from Cell Signaling (Boston, MA), Selleck (Houston, TX) and Tocris Bioscience (Bristol, UK), respectively. Compounds were dissolved in DMSO and used in vitro at a concentration indicated in the Figures. Cell culture media was replaced every 24 h. FACS For the separation of prostate cell lineages, dissociated murine prostate cells were stained with FITC- or Pacific blue-anti CD31,CD45 and Ter119 antibodies (eBioscience, San Diego, CA), PE-or PE-Cy7-anti Sca-1 antibody (eBioscience, San Diego, CA) and Alexa 647-anti CD49f antibody (Biolegend, San Diego, CA). FACS analyses and sorting were performed by using the BD LSR II or BD LSR Fortessa and Aria I, respectively (BD Biosciences). RNA isolation and qRT–PCR Total RNA was isolated from cells using the RNeasy Plus mini kit (Qiagen, Valencia, CA). Reverse transcription was performed using the iScript cDNA synthesis kit (Bio-Rad). qRT–PCR was performed using the SYBR Premix Ex Taq (Perfect Real Time; Takara Bio Inc., Otsu, Shiga, Japan) on a StepOne plus Real-Time PCR system (Applied Biosystems, Foster City, CA). Primer sequences for qPCR are listed in Supplementary Table 2 . Luciferase assay Three milligrams of D-luciferin (Promega, Madison, WI) in 100 μl phosphate-buffered saline was intraperitoneally injected to 8–12-week-old NICD WT :NF-kB-RE-Luc and PB- NICD;NF-kB-RE-Luc. After 10 min, prostates were harvested and bioluminescence imaging was performed with IVIS 200 (Caliper Life Sciences, Mountain View, CA). Imaged signals were quantitatively analysed with IGOR-PRO Living Image software (Caliper Life Sciences). Luciferase assay was performed using the Luciferase Reporter Assay System (Promega). Luciferase activity was normalized by total cell numbers or tissue weight. Adenovirus infection Dissociated primary prostate cells were infected with Ad5-CMV or Ad5-CMV-Cre (Viral Vector Production Core Laboratory, Baylor College of Medicine, Houston, TX) at an multiplicity of infection (MOI) of 50 at 37 °C for 1 h in DMEM. Cells were washed twice with DMEM and resuspended in PrEGM media to be used in the prostate sphere assay. Western blot Prostate tissues were lysed in RIPA buffer (20 mM Tris-HCl, pH 7.5, 150 mM NaCl, 1 mM Na 2 EDTA, 1 mM EGTA, 1% NP-40, 1% sodium deoxycholate, 2.5 mM sodium pyrophosphate, 1 mM β-glycerophosphate and 1 mM Na 3 VO 4 ) with protease inhibitors and phosphatase inhibitors (Roche Applied Science) using Tissuelyser LT (Qiagen). Protein concentrations were determined by a Bradford Assay kit (Bio-Rad). Protein was separated by 8 or 12% SDS/PAGE and transferred onto a polyvinylidene difluoride (PVDF) membrane (Amersham Biosciences, Arlington Heights, IL). The membrane was blocked in 5% skim milk, and subsequently incubated with primary antibodies listed in Supplementary Table 3 at 4 °C overnight followed by incubation with peroxidase-conjugated goat anti-mouse IgG or goat anti-rabbit IgG (Jackson ImmunoResearch, Inc., West Grove, PA), and developed with Pierce ECL reagent (Thermo Scientific, Rockford, IL). Reverse-phase protein array RPPAs were performed and analysed by the RPPA core of the MD Anderson Cancer Center. In brief, protein lysates obtained from primary samples were printed onto slides, together with normalization and expression controls, in five serial dilutions. The slides were probed with strictly validated primary antibodies against total or phosphorylated protein and a secondary antibody was used to amplify the signal. The stained slides were scanned using a scanner and the images were analysed using the MicroVigene Version 3.4 software programme (VigeneTech) to produce quantified data. The ‘supercurve’ algorithm was used to estimate the sample-specific protein expression levels. The RPPA data were normalized by median centring the results for each sample across all antibodies. Histology and immunostaining H&E staining and immunofluorescence staining were performed using standard protocols on 5-μm paraffin sections. Primary antibodies and dilutions used are listed in the Supplementary Table 3. Slides were incubated with 5% normal goat serum (Vector Labs) and with primary antibodies diluted in 2.5% normal goat serum overnight at 4 °C. Slides then were incubated with secondary antibodies (diluted 1:500 in 0.05% Tween 20 in phosphate-buffered saline (PBST)) labelled with Alexa Fluor 488 or 594 (Invitrogen/Molecular Probes). Sections were counterstained with 4',6-diamidino-2-phenylindole (Sigma-Aldrich). Immunofluorescence staining was imaged using an Olympus BX60 fluorescence microscope or a Leica EL6000 confocal microscope. Images of IHC were analysed by Image-Pro Plus version 6.3 by Media Cybernetics. Cell number was determined by using the count feature in the software that asks for the user to indicate the colour that would be used to indicate a positive cell. (For example: blue would be indicated to count nuclei and thus indicate total numbers of cells). Borders were created such that only epithelial cells would be analysed. Expression microarray Expression microarray assays were performed using 4 × 44 K Whole Mouse Genome Oligo Microarray chip (Agilent Technologies, Santa Clara, CA) and the Feature Extraction Software v9.1.3.1 (Agilent Technologies) was used to extract and analyse the signals. Statistics All experiments were performed using 2–8 mice in independent experiments. Data are presented as mean±s.d. Student’s t -test was used to determine significance between groups. For all statistical tests, the 0.05 level of confidence was accepted for statistical significance. One-sided Fisher’s exact tests also assessed enrichment between genes high in our PB-NICD group (544 unique genes with P <0.01, fold difference >1.5) and genes high in Akt or NF-κB signatures (710 and 270 genes, respectively). How to cite this article: Kwon, O.-J. et al . Increased Notch signalling inhibits anoikis and stimulates proliferation of prostate luminal epithelial cells. Nat. Commun. 5:4416 doi: 10.1038/ncomms5416 (2014). Accession codes: Array data have been deposited in Gene Expression Omnibus under accession number GSE53036 .